USE1 is a bispecific conjugating enzyme for ubiquitin and FAT10, which FAT10ylates itself incis The ubiquitin-like modifier FAT10 targets proteins for degradation by the proteasome and is activated by the E1 enzyme UBA6. In this study, we identify the UBA6-specific E2 enzyme (USE1) as an interaction partner of FAT10. Activated FAT10 can be transferred from UBA6 onto USE1 in vitro , and endogenous USE1 and FAT10 can be coimmunoprecipitated from intact cells. Small interfering RNA-mediated downregulation of USE1 mRNA resulted in a strong reduction of FAT10 conjugate formation under endogenous conditions, suggesting that USE1 is a major E2 enzyme in the FAT10 conjugation cascade. Interestingly, USE1 is not only the first E2 enzyme but also the first known substrate of FAT10 conjugation, as it was efficiently auto-FAT10ylated in cis but not in trans . The covalent conjugation with modifiers of the ubiquitin family is a versatile and widely used posttranslational modification that may change the function, fate or localization of specific target proteins. The formation of an isopeptide bond between the C terminus of ubiquitin and a lysine residue in a target protein requires the C-terminal glycine residue of ubiquitin to become activated by an E1-type enzyme that first adenylates ubiquitin and then transfers it onto a cysteine residue of the E1 enzyme to form a thioester. The activated ubiquitin is subsequently passed onto a cysteine in the active site of a ubiquitin-conjugating enzyme (E2). The ubiquitin-charged E2 enzyme and a specific substrate protein are then both bound by a ubiquitin ligase (E3) that catalyses the transfer of the activated ubiquitin onto the substrate protein [1] . In humans, there are dozens of E2 enzymes and hundreds of E3 enzymes, the specificity of which ensures that ubiquitylation is a highly regulated and substrate selective event. The initial activation of ubiquitin was for decades believed to be accomplished solely by a single enzyme designated as UBE1 [2] , [3] , until recently when it was shown that a second E1-type enzyme, called UBA6 (UBE1L2, E1-L2, MOP-4), exists, which can also activate ubiquitin [4] , [5] , [6] . Interestingly, UBE1 and UBA6 do not cooperate with the same set of E2 enzymes and one E2 enzyme has been described that can accept ubiquitin only from UBA6 but not from UBE1. This E2 enzyme, which was originally named E2Z [7] , has accordingly been renamed as UBA6-specific E2 enzyme (USE1) [5] . The principle of ubiquitin activation and conjugation by an E1–E2–E3 cascade also applies to several well-investigated ubiquitin-like modifiers including SUMO-1/2/3, NEDD8, ISG15 and ATG8/12. Each of these subfamilies of modifiers uses their private E1, E2 and E3 enzymes to ensure that a unique modifier is specifically transferred through the respective private E2 and E3 enzymes onto the correct target substrate [8] , [9] . This elaborate specificity allows separate regulation of conjugation with each of the known ubiquitin-like modifiers and it ensures that a given substrate is not derivatized by the wrong modifier. This principle of wholly specific enzymes was found to be violated when it was discovered recently that the E1 enzyme UBA6 activates not only ubiquitin but also the ubiquitin-like modifier FAT10 [6] . This finding poses the interesting question of how this E1 enzyme can discriminate between an E2 enzyme that needs to be charged with activated ubiquitin or FAT10 [10] . As E2 enzymes Ubc5 and Ubc13 can be charged with activated ubiquitin but not with FAT10 in vitro [6] , it is possible that the discrimination between ubiquitin and FAT10 may occur at the level of E2 enzymes. FAT10 is an interferon (IFN)γ- and tumour necrosis factor (TNF)α-inducible ubiquitin-like modifier that is encoded in the major histocompatibility complex class I locus and is constitutively expressed in mature dendritic cells and B cells [11] , [12] , [13] . FAT10 consists of two ubiquitin-like domains in tandem array and bears a free diglycine motif at its C terminus, which is required for the covalent conjugation to as yet unidentified target proteins [6] , [14] . The biological function of FAT10 remains poorly understood, but it has been shown that overexpression of FAT10 leads to caspase-dependent apoptosis in a mouse fibroblast cell line [13] and renal tubular epithelial cells [15] . In addition, FAT10 has been shown to serve as a signal for proteasomal degradation independently of the ubiquitylation system [16] , [17] . NEDD8 ultimate buster long (NUB1L), a cytokine-inducible linker protein that non-covalently interacts with FAT10 through its three C terminal ubiquitin-associated (UBA) domains and with the 26S proteasome through its N-terminal ubiquitin-like (UBL) domain, accelerates the degradation of FAT10 and FAT10-linked proteins [18] , [19] . In this study, we sought to further characterize the conjugation pathway of FAT10. Stimulated by the identification of USE1 as an interaction partner of FAT10 in a yeast two-hybrid screening assay, we characterized USE1 as a conjugating enzyme for FAT10 in vitro and in vivo . Interestingly, USE1 turned out to be not only a major E2 enzyme for FAT10 but also the first substrate of FAT10, as USE1 was demonstrated to auto-Fat10ylate itself in cis . Identification USE1 as an interaction partner of FAT10 It has recently been shown that UBA6 is an E1 enzyme not only for ubiquitin but also for FAT10 [6] . During in vitro activation experiments, we had obtained independent evidence that UBA6 can activate FAT10; however, in some of the experiments, an activation of FAT10 by UBE1L was also observed (C. Pelzer, unpublished data). To further investigate the interaction between these E1 enzymes and FAT10, a yeast two-hybrid assay was performed. FAT10 could only interact with UBA6, but not with the closely related E1-type enzymes UBE1 and UBE1L, whereas ISG15, used as control, interacted specifically with UBE1L, but not with UBE1 or UBA6 ( Fig. 1 ). The interaction between the proteins described was clear in an 5-bromo-4-chloro-3-indolyl-β- D -galactoside (X-Gal) filter assay and as judged from the colour change on selective growth plates. Therefore, our data are consistent with UBA6 being the E1 enzyme for FAT10, as ISG15, which has a similar structure as the one predicted for FAT10 [10] , [20] , cannot interact with UBA6. 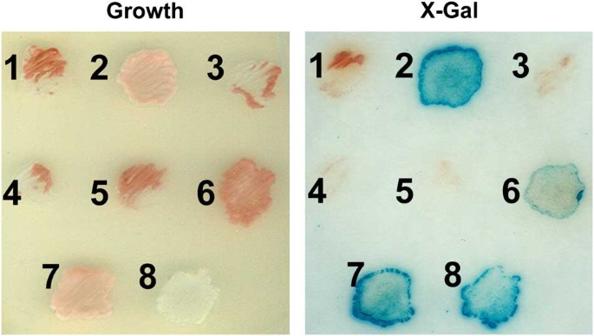Figure 1: FAT10 interacts specifically with UBA6 and USE1 in yeast two-hybrid assays. Yeast NMY51 was co-transformed with pLexA-N-ISG15 and pACT2-UBE1 (1), with pACT2-UBE1L (2) or pACT2-UBA6 (3), respectively, or with pLexA-FAT10 and pACT2-UBE1 (4), pACT2-UBE1L (5), pACT2-UBA6 (6), pACT2-USE1short (7) or pACT2-USE1 full length (8), respectively, and grown on 3-AT-containing selection plates lacking tryptophan, leucine and histidine (left panel). An X-Gal filter assay was performed to verify the interaction of the respective proteins (right panel). A representative experiment from a total of three experiments with similar outcome is shown. Figure 1: FAT10 interacts specifically with UBA6 and USE1 in yeast two-hybrid assays. Yeast NMY51 was co-transformed with pLexA-N-ISG15 and pACT2-UBE1 (1), with pACT2-UBE1L (2) or pACT2-UBA6 (3), respectively, or with pLexA-FAT10 and pACT2-UBE1 (4), pACT2-UBE1L (5), pACT2-UBA6 (6), pACT2-USE1short (7) or pACT2-USE1 full length (8), respectively, and grown on 3-AT-containing selection plates lacking tryptophan, leucine and histidine (left panel). An X-Gal filter assay was performed to verify the interaction of the respective proteins (right panel). A representative experiment from a total of three experiments with similar outcome is shown. Full size image To identify a possible E2 enzyme for FAT10, a yeast two-hybrid screen was performed, with human FAT10 serving as a bait for screening of a human thymus library. This approach was chosen, as it has been shown previously that, at least in some cases, E2 enzymes can non-covalently interact directly with their cognate ubiquitin-like modifiers [21] . Sequencing of positive clones revealed that, besides the known interaction partner NUB1L [18] , a truncated version of E2 enzyme USE1 was among the identified putative interaction partners of FAT10. This result was further pursued because USE1 has been shown to take over activated ubiquitin from UBA6 [5] , the E1 enzyme of FAT10 [6] , and because we could show by yeast two-hybrid interaction assay that USE1 specifically interacted with UBA6 but not with UBE1 or UBE1L ( Supplementary Fig. S1 and Supplementary note online). The isolated cDNA of USE1 lacked 259 nucleotides at the 5′ end, designated USE1short. Hence, it was necessary to also test full-length USE1, which is extended N terminally [5] . The complete USE1 cDNA was therefore cloned into the prey vector and a yeast two-hybrid assay was carried out again. The full-length USE1 also resulted in a blue colour change in the X-Gal filter assay, demonstrating the interaction of the proteins ( Fig. 1 , right panel). In addition to the growth on the selection plates already indicating the interaction of FAT10 and USE1 the cotransformants showed a colour change to faint pink for USE1short or to white for full-length USE1 ( Fig. 1 , left panel). From the difference in colour, it seemed that full-length USE1 interacts more strongly with FAT10. Thus, we concluded that both USE1short and the full-length USE1 interact with FAT10 under the conditions in the yeast two-hybrid assay and we hypothesized that USE1 might function as an E2 enzyme for FAT10. USE1 serves as a conjugating enzyme for FAT10 in vitro and in vivo To test in vitro whether the transfer of FAT10 onto USE1 can occur, in vitro- transcribed and -translated FLAG-His-FAT10 or FLAG-His-FAT10ΔGG was incubated with recombinant His-tagged USE1 in the presence of recombinant glutathione- S -transferase (GST)-UBA6. The in vitro conjugation assay revealed that FAT10 was covalently linked to USE1 and the amount of FAT10-charged GST-UBA6 decreased simultaneously ( Fig. 2a ). FLAG-His-FAT10ΔGG served as a negative control, and was not transferred onto His-USE1 protein. Similar experiments conducted with ubiquitin ( Fig. 2b ) showed that haemagglutinin (HA)-tagged ubiquitin readily conjugated to USE1 in accordance with a previous report [5] . These results indicate that USE1 is not exclusively a conjugating enzyme for ubiquitin but also serves as an E2 enzyme for FAT10 in vitro . 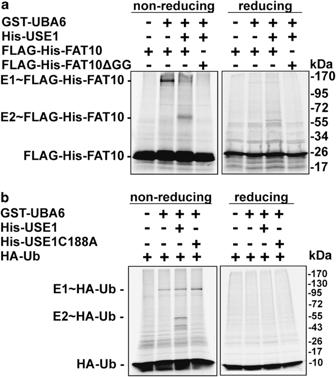Figure 2: FAT10 is transferred from UBA6 onto USE1in vitro. (a) Bacterially expressed affinity-purified His-USE1 was incubated together with adenosine triphosphate (ATP), recombinant GST-UBA6 andin vitrotranscribed and translated35S-labelled FLAG-His-FAT10 bound to anti-FLAG beads (lane 3 from the left). As negative controls, FLAG-His-FAT10 alone (lane 1), FLAG-His-FAT10 and GST-UBA6 (lane 2), and FLAG-His-FAT10ΔGG with GST-UBA6 and His-USE1 (lane 4) were used. Samples were subjected to non-reducing (left) and reducing (right) SDS–polyacrylamide gel electrophoresis (PAGE) and visualized by autoradiography. The positions of FAT10, the FAT10–USE1 conjugate (E2∼Flag-His-FAT10) and the FAT10–UBA6 conjugate (E1∼Flag-His-FAT10) are indicated at the left. (b) As a control, bacterially expressed affinity-purified His-USE1 was incubated, together with ATP, recombinant GST-UBA6 andin vitro-transcribed and -translated35S-labelled HA-ubiquitin bound to anti-HA beads (lane 3 from the left). As negative controls, HA-ubiquitin alone (lane 1), HA-ubiquitin with GST-UBA6 (lane2) or HA-ubiquitin with GST-UBA6 and His-[C188A]USE1 (lane 4) were used. Samples were subjected to non-reducing (left) and reducing (right) SDS–PAGE and visualized by autoradiography. The positions of HA-ubiquitin, the ubiquitin-USE1 conjugate (E2∼HA-ubiquitin) and the ubiquitin-UBA6 conjugate (E1∼HA-ubiquitin) are indicated on the left. The experiments shown are one out of three experiments performed with similar outcome. Figure 2: FAT10 is transferred from UBA6 onto USE1 in vitro . ( a ) Bacterially expressed affinity-purified His-USE1 was incubated together with adenosine triphosphate (ATP), recombinant GST-UBA6 and in vitro transcribed and translated 35 S-labelled FLAG-His-FAT10 bound to anti-FLAG beads (lane 3 from the left). As negative controls, FLAG-His-FAT10 alone (lane 1), FLAG-His-FAT10 and GST-UBA6 (lane 2), and FLAG-His-FAT10ΔGG with GST-UBA6 and His-USE1 (lane 4) were used. Samples were subjected to non-reducing (left) and reducing (right) SDS–polyacrylamide gel electrophoresis (PAGE) and visualized by autoradiography. The positions of FAT10, the FAT10–USE1 conjugate (E2 ∼ Flag-His-FAT10) and the FAT10–UBA6 conjugate (E1 ∼ Flag-His-FAT10) are indicated at the left. ( b ) As a control, bacterially expressed affinity-purified His-USE1 was incubated, together with ATP, recombinant GST-UBA6 and in vitro- transcribed and -translated 35 S-labelled HA-ubiquitin bound to anti-HA beads (lane 3 from the left). As negative controls, HA-ubiquitin alone (lane 1), HA-ubiquitin with GST-UBA6 (lane2) or HA-ubiquitin with GST-UBA6 and His-[C 188 A]USE1 (lane 4) were used. Samples were subjected to non-reducing (left) and reducing (right) SDS–PAGE and visualized by autoradiography. The positions of HA-ubiquitin, the ubiquitin-USE1 conjugate (E2 ∼ HA-ubiquitin) and the ubiquitin-UBA6 conjugate (E1 ∼ HA-ubiquitin) are indicated on the left. The experiments shown are one out of three experiments performed with similar outcome. Full size image To further characterize the interaction between FAT10 and USE1 in vivo , coimmunoprecipitation experiments were conducted in transiently transfected HEK293 cells. A higher-molecular-weight conjugate between HA-FAT10 and 6His-USE1 could be detected by western blot analysis under either reducing or non-reducing conditions, which was not observed when the catalytic site Cys 188 of USE1 was mutated to alanine ( Fig. 3a ). When His-USE1 and HA-ubiquitin were coexpressed, a His-USE1 ∼ HA-Ub conjugate could be readily detected under non-reducing conditions but, in contrast to the His-USE1-HA-FAT10 conjugate, it could be cleaved readily with β-mercaptoethanol, consistent with thioester linkage ( Fig. 3b ). As a control, we performed similar experiments with UbcH8, which can serve as a conjugating enzyme both for ISG15 and ubiquitin in vitro [22] , [23] , [24] . In contrast to USE1, UbcH8 did not form a conjugate with FAT10, but only with ubiquitin under non-reducing conditions ( Fig. 3c ). When these samples were treated with reducing agents, the interaction disappeared. Therefore, FAT10 cannot be transferred to UbcH8, but to USE1, forming a covalent and non-reducible bond in vivo . 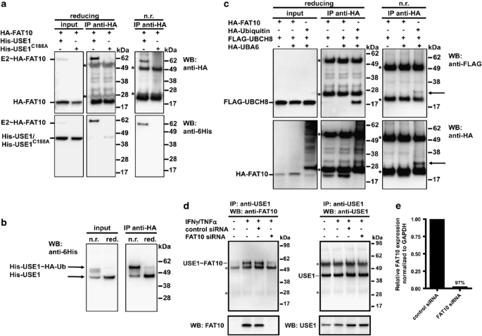Figure 3: Conjugate formation of FAT10 and USE1in vivo. (a) Coimmunoprecipitation of HA-FAT10 and His6-USE1. HEK293 cells were transiently transfected with pcDNA3.1-HA-FAT10 and pcDNA3.1/His-A-Xpress-USE1, as indicated. After immunoprecipitation against the HA-tag of FAT10, samples were subjected to western analysis with a peroxidase-conjugated polyhistidine-reactive antibody or an HA-reactive mAb. Samples were analysed under non-reducing (n.r.) and reducing conditions. (b) Coimmunoprecipitation of HA-ubiquitin and His6-USE1. HEK293 cells were transfected with pcDNA3.1-HA-ubiquitin and pcDNA3.1/His-A-Xpress-USE1. After immunoprecipitation against the HA-tag of HA-ubiquitin, samples were subjected to western blot analysis with a peroxidase-conjugated polyhistidine-reactive antibody. Samples were analysed under n.r. and reducing (red.) conditions. (c) Coimmunoprecipitation from HA-FAT10-, HA-ubiquitin (Ub)-, FLAG-UbcH8- or HA-UBA6-expressing cells, which were transiently transfected with pcDNA3.1-HA-FAT10, pcDNA3.1-HA-Ub, pcDNA3-FLAG-UBCH8 or pcDNA3.1-HA-UBA6 as indicated. After immunoprecipitation with anti-HA-Sepharose, reduced and n.r. samples were subjected to western blot analysis with HA-reactive and FLAG-reactive mAb. Asterisks indicate the heavy and light chains of the HA-reactive antibody used for the immunoprecipitation. Arrows indicate the FLAG-UbcH8-HA-Ub conjugate. Representative experiments out of three experiments with similar outcome are shown. (d) Coimmunoprecipitation of endogeneous USE1 and FAT10 from HEK293 cells. Cells were transfected twice with a negative control siRNA or with a mixture of four siRNAs against FAT10 and subsequently treated with 200 U ml−1IFNγ and 400 U ml−1TNFα. After 3 days, cells were lysed and USE1 was immunoprecipitated using a USE1-reactive rabbit mAb. Subsequently, proteins were subjected to western blot analysis using a FAT10-reactive mAb (left panel) or a USE1-reactive mAb (right panel) under reducing conditions. Loading controls are shown in the bottom panels. (e) The knockdown of FAT10 was confirmed by real-time RT–PCR. The relative FAT10 mRNA expression level in IFNγ/TNFα-treated HEK293 cells transfected with control siRNA was set to unity and RNA levels were normalized to the expression of glyceraldehyde-3-phosphate dehydrogenase. The experiments have been repeated three times with similar outcome. Asterisks indicate the heavy and light chains of the HA-reactive antibody used for the immunoprecipitation. Figure 3: Conjugate formation of FAT10 and USE1 in vivo . ( a ) Coimmunoprecipitation of HA-FAT10 and His 6 -USE1. HEK293 cells were transiently transfected with pcDNA3.1-HA-FAT10 and pcDNA3.1/His-A-Xpress-USE1, as indicated. After immunoprecipitation against the HA-tag of FAT10, samples were subjected to western analysis with a peroxidase-conjugated polyhistidine-reactive antibody or an HA-reactive mAb. Samples were analysed under non-reducing (n.r.) and reducing conditions. ( b ) Coimmunoprecipitation of HA-ubiquitin and His 6 -USE1. HEK293 cells were transfected with pcDNA3.1-HA-ubiquitin and pcDNA3.1/His-A-Xpress-USE1. After immunoprecipitation against the HA-tag of HA-ubiquitin, samples were subjected to western blot analysis with a peroxidase-conjugated polyhistidine-reactive antibody. Samples were analysed under n.r. and reducing (red.) conditions. ( c ) Coimmunoprecipitation from HA-FAT10-, HA-ubiquitin (Ub)-, FLAG-UbcH8- or HA-UBA6-expressing cells, which were transiently transfected with pcDNA3.1-HA-FAT10, pcDNA3.1-HA-Ub, pcDNA3-FLAG-UBCH8 or pcDNA3.1-HA-UBA6 as indicated. After immunoprecipitation with anti-HA-Sepharose, reduced and n.r. samples were subjected to western blot analysis with HA-reactive and FLAG-reactive mAb. Asterisks indicate the heavy and light chains of the HA-reactive antibody used for the immunoprecipitation. Arrows indicate the FLAG-UbcH8-HA-Ub conjugate. Representative experiments out of three experiments with similar outcome are shown. ( d ) Coimmunoprecipitation of endogeneous USE1 and FAT10 from HEK293 cells. Cells were transfected twice with a negative control siRNA or with a mixture of four siRNAs against FAT10 and subsequently treated with 200 U ml −1 IFNγ and 400 U ml −1 TNFα. After 3 days, cells were lysed and USE1 was immunoprecipitated using a USE1-reactive rabbit mAb. Subsequently, proteins were subjected to western blot analysis using a FAT10-reactive mAb (left panel) or a USE1-reactive mAb (right panel) under reducing conditions. Loading controls are shown in the bottom panels. ( e ) The knockdown of FAT10 was confirmed by real-time RT–PCR. The relative FAT10 mRNA expression level in IFNγ/TNFα-treated HEK293 cells transfected with control siRNA was set to unity and RNA levels were normalized to the expression of glyceraldehyde-3-phosphate dehydrogenase. The experiments have been repeated three times with similar outcome. Asterisks indicate the heavy and light chains of the HA-reactive antibody used for the immunoprecipitation. Full size image Formation of a USE1–FAT10 conjugate in cytokine-stimulated cells To test whether a USE1–FAT10 conjugate can also be found in the absence of overexpression, we treated HEK293 cells with TNF-α and IFN-γ to induce FAT10 and then performed immunoprecipitation with a rabbit monoclonal anti-USE1 antibody, followed by western blot analysis with either a newly generated FAT10-specific monoclonal antibody (mAb) (designated 4F1, see Supplementary Fig. S3 online) or a USE1-specific mAb under reducing conditions (10% 2-ME). The blots shown in Fig. 3d reveal that the endogenous FAT10–USE1 conjugate was detectable in the presence but not in the absence of FAT10 induction by proinflammatory cytokines (anti-FAT10 blot, lanes 1 and 2). Consistently, the endogeneous conjugate was strongly diminished when FAT10 was downregulated by FAT10-specific small interfering RNA (siRNA) but not when cells were treated with a negative control siRNA (anti-FAT10 blot, lanes 3 and 4). The successful knockdown of FAT10 mRNA by about 97%, compared with treatment with control siRNA, was verified by real-time reverse transcription (RT)–PCR ( Fig. 3e ). When USE1 was immunoprecipitated with USE1-specific mAb, followed by western analysis with the same USE1-specific mAb ( Fig. 3d , right panel) or a USE1-specific pAb (data not shown), we failed to visualize the endogenous USE1–FAT10 conjugate in most experiments, as this detection system was not sensitive enough for this purpose. To address the question of the relevant efficiency of charging USE1 with ubiquitin versus FAT10, a semiendogenous immunoprecipitation experiment was performed, in which, on transfection of HEK293 cells with expression constructs for FLAG-His-USE1 and HA-ubiquitin, FAT10 expression was induced with IFNγ and TNFα. As shown in Supplementary Fig. S5 , the USE1–FAT10 conjugate was clearly formed next to the USE1–Ub conjugate (IP, lane 4). In cells that expressed HA-ubiquitin, the USE1–FAT10 conjugate was still readily detectable, indicating that endogenous FAT10 could compete with ubiquitin for conjugation to USE1 (IP, lane 5 versus 4). Under reducing conditions, the USE1–ubiquitin conjugate was completely reduced, whereas the USE1–FAT10 conjugate was not (data not shown). Silencing of USE1 leads to a reduction of FAT10 conjugates To determine whether USE1 has a central role in FAT10 conjugate formation in vivo , we tested whether targeted knockdown of USE1 with siRNA leads to a significant reduction of FAT10 conjugates in HEK293 cells transfected with a FLAG-His-FAT10 expression construct. As a control, knockdown of UBA6 or UBA6 and USE1 together was performed. Immunoprecipitation experiments in Fig. 4a showed that the downregulation of endogenous USE1 by about 90% as measured by real-time RT–PCR ( Fig. 4b ), compared with HEK293 cells transfected with control siRNA, led to a strong decrease in the amount of FAT10 conjugates, which was comparable to the decrease of FAT10 conjugates observed with a 90% downregulation of UBA6 mRNA. This effect was slightly enhanced when both USE1 and UBA6 were downregulated simultaneously. As a control, cells were transfected with the diglycine mutant of FAT10 (FLAG-His-FAT10ΔGG) that did not show FAT10 conjugation. As a loading control for the prepared lysates, β-actin was used for western blot analysis and the levels of UBA6, USE1 and FLAG-His-FAT10 proteins in the lysates used for immunoprecipitation were monitored by western blot analysis ( Fig. 4a , lower panels). As transfection of cells with siRNA also lowered the total amount of monomeric FAT10 in the cells, we quantified enhance chemiluminescence signals with Quantity One Software (BioRad) and calculated a coefficient of conjugated FAT10:mono-FAT10, which was 1.0 for lane 2 (no siRNA), 0.96 for lane 3 (control siRNA), 0.4 for lane 4 (UBA6 siRNA), 0.7 for lane 5 (USE1 siRNA), 0.5 for lane 6 (UBA6 and USE1 siRNA) and 0.04 for lane 7 (diglycine mutant of FAT10), clearly showing the reduction of FAT10 conjugates after downregulation of USE1 or UBA6. To exclude off-target effects by using a mixture of four different USE1 siRNAs, each single siRNA was used separately to downregulate USE1 in HEK293 cells, which also led to a clear reduction of FAT10 conjugates ( Supplementary Fig. S6 online), further supporting the results shown in Fig. 4a . 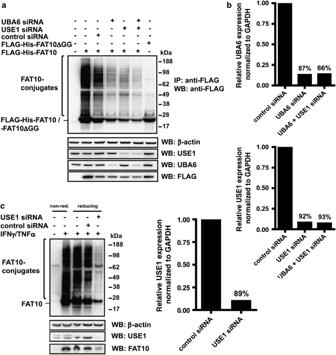Figure 4: Knockdown of USE1 leads to impaired FAT10 conjugate formation. (a) HEK293 cells were either transfected or not transfected with a mixture of four different siRNAs against UBA6, USE1, both together or with a control siRNA, and subsequently transfected with an expression plasmid encoding FLAG-His-FAT10 or its diglycine mutant FLAG-His-FAT10ΔGG. After 4 days, an anti-FLAG immunoprecipitation was performed and the precipitates were analysed by western blot using a directly peroxidase-linked anti-FLAG mAb to evaluate FAT10 conjugate formation. Untransfected HEK293 cells or HEK293 cells transfected with FLAG-His-FAT10 or its mutant form, FLAG-His-FAT10ΔGG, served as positive or negative control for the FAT10-conjugate formation, respectively. In the upper panel, the western blot against FLAG-FAT10 after the immunoprecipitation of FLAG-FAT10 conjugates is shown. The lower panels show the expression levels of USE1, UBA6 and FAT10, respectively; β-actin served as a loading control for the western blot. (b) The knockdown of USE1 and UBA6 was confirmed by real-time RT–PCR. The relative UBA6 or USE1 mRNA expression level in HEK293 cells, transfected with control siRNA and FLAG-His-FAT10 was set to unity and RNA levels were normalized to the expression of glyceraldehyde-3-phosphate dehydrogenase. A representative experiment out of three with similar outcome is shown. (c) HEK293 cells were transfected twice with siRNA against USE1 and subsequently treated for 24 h with IFNγ/TNFa to induce endogenous FAT10 expression, followed by an immunoprecipitation using a FAT10-specific mAb. FAT10 conjugates were analysed on a western blot using a FAT10 pAb (left panel). Knockdown of USE1 (right panel) was confirmed by real-time RT–PCR as described in (b). One out of three experiments with similar outcome is shown. Figure 4: Knockdown of USE1 leads to impaired FAT10 conjugate formation. ( a ) HEK293 cells were either transfected or not transfected with a mixture of four different siRNAs against UBA6, USE1, both together or with a control siRNA, and subsequently transfected with an expression plasmid encoding FLAG-His-FAT10 or its diglycine mutant FLAG-His-FAT10ΔGG. After 4 days, an anti-FLAG immunoprecipitation was performed and the precipitates were analysed by western blot using a directly peroxidase-linked anti-FLAG mAb to evaluate FAT10 conjugate formation. Untransfected HEK293 cells or HEK293 cells transfected with FLAG-His-FAT10 or its mutant form, FLAG-His-FAT10ΔGG, served as positive or negative control for the FAT10-conjugate formation, respectively. In the upper panel, the western blot against FLAG-FAT10 after the immunoprecipitation of FLAG-FAT10 conjugates is shown. The lower panels show the expression levels of USE1, UBA6 and FAT10, respectively; β-actin served as a loading control for the western blot. ( b ) The knockdown of USE1 and UBA6 was confirmed by real-time RT–PCR. The relative UBA6 or USE1 mRNA expression level in HEK293 cells, transfected with control siRNA and FLAG-His-FAT10 was set to unity and RNA levels were normalized to the expression of glyceraldehyde-3-phosphate dehydrogenase. A representative experiment out of three with similar outcome is shown. ( c ) HEK293 cells were transfected twice with siRNA against USE1 and subsequently treated for 24 h with IFNγ/TNFa to induce endogenous FAT10 expression, followed by an immunoprecipitation using a FAT10-specific mAb. FAT10 conjugates were analysed on a western blot using a FAT10 pAb (left panel). Knockdown of USE1 (right panel) was confirmed by real-time RT–PCR as described in ( b ). One out of three experiments with similar outcome is shown. Full size image In a second approach, the USE1 knockdown experiment was conducted under completely endogeneous conditions. Therefore, cells were again transfected with siRNA against USE1 and subsequently endogeneous FAT10 expression was induced by stimulation of cells for 24 h with IFNγ/TNFα. As shown in Fig. 4c , knockdown of USE1 mRNA by about 89% as compared with control siRNA-transfected cells led to a strong reduction of FAT10 conjugates relative to FAT10 monomer expression under completely endogeneous conditions, with coefficients of conjugated FAT10: mono-FAT10 of 1 for lane 3 (no siRNA), 0.3 for lane 4 (control siRNA) and 0.1 for lane 5 (USE1 siRNA). USE1 auto-FAT10ylates itself in cis but not in trans In view of the fact that the USE1–FAT10 conjugate could not be reduced, we hypothesized that USE1 auto-FAT10ylates itself. To investigate this hypothesis, we generated expression constructs for HA-USE1 and an HA-tagged USE1 mutant in which all 11 lysines were replaced by arginines. Transient co-transfection of HEK293T cells with FLAG-His-FAT10 and with either HA-USE1 wild-type or HA-USE1 11K-11R mutant, followed by combined immunoprecipitation and western blot analysis, revealed that both wild-type USE1 and the 11K-11R mutant formed a conjugate with FLAG-His-FAT10 under non-reducing conditions, thus indicating that the mutant was functional for thioester formation ( Fig. 5 ). In contrast to the conjugate formed with the USE1 wild-type protein, FLAG-His-FAT10 ∼ HA-USE1-11K-11R could be largely reduced, suggesting that the two proteins are mainly thioester linked. Whether the residual complex was due to FAT10ylation of the USE1 N terminus or whether residues other than lysine were FAT10ylated or whether some thioester bonds resisted boiling in β-ME remains to be determined. 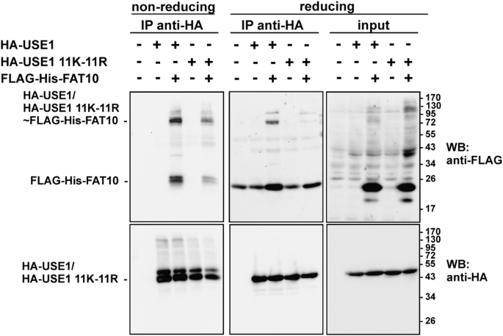Figure 5: Coimmunoprecipitation of HA-USE1 wild type or HA-USE1 11K-11R mutant with 3xFLAG-His-FAT10. As indicated above the panels, HEK293 cells were transiently co-transfected with pcDNA.3.1-3xFLAG-His-FAT10 and with either pcDNA3.1-HA-USE1 encoding USE1 wild type or pcDNA3.1-HA-USE1 11K-11R encoding a USE1 mutant in which all lysines were replaced by arginines. After anti-HA immunoprecipitation against USE1, samples were separated on SDS–polyacrylamide gel electrophoresis and subjected to western blot analysis with either FLAG-reactive antibody conjugated to horseradish peroxidase (HRP) (top panels) or HRP-conjugated HA-reactive antibody (bottom panels). Samples were analysed under non-reducing (left panels) and reducing conditions (right panels). A representative experiment out of three with similar outcome is shown. Figure 5: Coimmunoprecipitation of HA-USE1 wild type or HA-USE1 11K-11R mutant with 3xFLAG-His-FAT10. As indicated above the panels, HEK293 cells were transiently co-transfected with pcDNA.3.1-3xFLAG-His-FAT10 and with either pcDNA3.1-HA-USE1 encoding USE1 wild type or pcDNA3.1-HA-USE1 11K-11R encoding a USE1 mutant in which all lysines were replaced by arginines. After anti-HA immunoprecipitation against USE1, samples were separated on SDS–polyacrylamide gel electrophoresis and subjected to western blot analysis with either FLAG-reactive antibody conjugated to horseradish peroxidase (HRP) (top panels) or HRP-conjugated HA-reactive antibody (bottom panels). Samples were analysed under non-reducing (left panels) and reducing conditions (right panels). A representative experiment out of three with similar outcome is shown. Full size image To investigate whether auto-FAT10ylation occurs in cis or in trans , HEK293 cells were transfected with HA-FAT10 and with either His 6 -tagged USE1 wild-type or FLAG-His tagged [C 188 A]USE1 mutant alone, or in combination with both together. The outcome of the immunoprecipitation assays analysed by western blot was that His 6 -USE1 wild type only transferred FAT10 onto itself either with HA-FAT10 alone or in the setup in which the FLAG-His-USE1-[C 188 A] mutant was co-transfected. The inactive mutant did not form a conjugate when it was coexpressed with just HA-FAT10 and also not when active and inactive USE1 and HA-FAT10 were coexpressed ( Fig. 6 ). Therefore, auto-FAT10ylation of USE1 occurs in cis but not in trans . 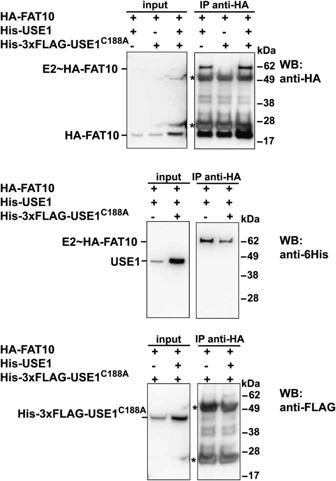Figure 6: USE1 transfers FAT10 incisbut not intrans. Coimmunoprecipitation of HA-FAT10- and His6-USE1 and 3xFLAG-His6-[C188A]USE1-expressing HEK293 cells. Cells were transiently transfected with pcDNA3.1-HA-FAT10 and pcDNA3.1/His-A-Xpress-USE1 or pcDNA3.1-3xFLAG-His6-[C188A]USE1, as indicated above the top panel. After immunoprecipitation against the HA-tag of FAT10, samples were separated on 4–12% bis-Tris SDS gels and subjected to western blot analysis with an HA-reactive monoclonal antibody (top panel), a peroxidase-conjugated polyhistidine reactive antibody (middle panel) or a FLAG M2-reactive mAb (bottom panel). Asterisks indicate the heavy and light chains of the HA-reactive antibody used for the immunoprecipitation. The positions of the USE1∼HA-FAT10 conjugate (E2∼HA-FAT10), HA-FAT10, His-USE1 and FLAG-[C188A]USE1 are indicated on the left. A representative experiment out of three experiments with similar outcome is shown. Figure 6: USE1 transfers FAT10 in cis but not in trans . Coimmunoprecipitation of HA-FAT10- and His 6 -USE1 and 3xFLAG-His 6 -[C 188 A]USE1-expressing HEK293 cells. Cells were transiently transfected with pcDNA3.1-HA-FAT10 and pcDNA3.1/His-A-Xpress-USE1 or pcDNA3.1-3xFLAG-His 6 -[C 188 A]USE1, as indicated above the top panel. After immunoprecipitation against the HA-tag of FAT10, samples were separated on 4–12% bis-Tris SDS gels and subjected to western blot analysis with an HA-reactive monoclonal antibody (top panel), a peroxidase-conjugated polyhistidine reactive antibody (middle panel) or a FLAG M2-reactive mAb (bottom panel). Asterisks indicate the heavy and light chains of the HA-reactive antibody used for the immunoprecipitation. The positions of the USE1 ∼ HA-FAT10 conjugate (E2 ∼ HA-FAT10), HA-FAT10, His-USE1 and FLAG-[C 188 A]USE1 are indicated on the left. A representative experiment out of three experiments with similar outcome is shown. Full size image FAT10 is a very young member of the ubiquitin family, young in terms of evolution as it is found only in mammals, and young in terms of the history of investigation, beginning with its discovery in the histocompatibility complex class I locus in 1996 [25] . In this study, we identify an E2 enzyme for FAT10, as well as the first substrate of FAT10 conjugation, and show that it is the same protein, USE1. To identify new interaction partners of FAT10, we performed a yeast two-hybrid screen using a human thymus cDNA library, as FAT10 was found to be most highly expressed in the thymus [26] . Our screen identified 11 different bait-dependent clones, but USE1 was the only E2 enzyme found among these putative FAT10-interacting proteins. A priori one would not need to postulate a high affinity binding between a modifier and a cognate E2 enzyme. Nevertheless, it has recently been shown for SUMO-1 that it binds to its cognate E2 enzyme UBC9 not only through a thioester linkage but also non-covalently, and that this non-covalent interaction promotes the formation of short SUMO-1 chains [21] . Moreover, for ubiquitin, a non-covalent interaction with the heterodimeric E2 enzyme Mms2/Ubc13 has been shown [27] . A weak non-covalent interaction between FAT10 and USE1 was therefore a reasonable basis for investigating USE1 as a potential E2 enzyme for FAT10. Another striking argument for USE1 as a potential E2 enzyme for FAT10 was that USE1 was identified as the only E2 enzyme that could receive activated ubiquitin exclusively from UBA6 and not from UBE1 [5] . Moreover, it was shown that depletion of UBA6 but not of UBE1 reduced the charging of USE1 with activated ubiquitin in intact cells. Although these data convincingly document a functional cooperation between UBA6 and USE1, an interaction between these E1 and E2 enzymes has not been shown. By yeast two-hybrid screen, we show that UBA6 and USE1 indeed interact and that this interaction is specific and did not occur with UBE1 or UBE1L ( Supplementary Fig. S1 ). Combined with the identification of UBA6 as the E1 enzyme of FAT10 [6] , it was therefore clearly warranted to investigate USE1 as an E2 enzyme for FAT10 conjugation. By in vitro FAT10 transfer assays, we showed that radioactively labelled FAT10 was activated by UBA6. In the presence of USE1, the amount of UBA6 ∼ FAT10 was reduced and instead a complex of radioactive FAT10 bound to USE1 appeared ( Fig. 2a ). These data show that purified FAT10, UBA6 and USE1 are sufficient to generate FAT10-charged USE1 in vitro . The enzymatic transfer of FAT10 both to UBA6 and to USE1 in vitro relied on the C-terminal diglycine motif of FAT10, consistent with the formation of a thioester bond between the C terminus of FAT10 and the active-site cysteine residues of UBA6 and USE1. Whether the active-site cysteine of USE1 was indeed required for formation of a FAT10–USE1 conjugate was then investigated in coimmunoprecipitation experiments ( Fig. 3a ). Coexpression of FAT10 with wild-type USE1 resulted in the formation of a USE1–FAT10 conjugate in intact cells, but this was not the case when the [C 188 A]USE1 active-site mutant was used. Formation of such a conjugate was specific for USE1, as a similar coexpression experiment performed with UbcH8, which is a bispecific E2 enzyme for ubiquitin and ISG15 [22] , [23] , formed a conjugate with ubiquitin but not with FAT10 ( Fig. 3c ). To investigate whether USE1 is in fact required for FAT10 conjugation to target proteins, USE1 expression was downregulated by siRNA transfection of HEK293 cells transiently expressing FLAG-FAT10 and also in TNF-α/IFN-γ-stimulated HEK293 cells. Using our newly generated FAT10-reactive mAb for immunoprecipitation, we could show for the first time that endogenously expressed FAT10 forms a broad high-molecular-weight smear of bona fide FAT10 conjugates that were only observed after FAT10 induction by proinflammatory cytokines. Interestingly, siRNA-mediated reduction of USE1 mRNA expression by 92% led to a strong decrease in the intensity of conjugate bands ( Fig. 4 ). A pretreatment with siRNA in general reduced the amount of transiently expressed FAT10, which was probably due to a reduced transfection efficiency ( Fig. 4a ). The siRNAs specific for UBA6 or USE1 strongly reduced FAT10 conjugates but, unexpectedly, also to some extent monomeric FAT10. We repeatedly observed that silencing of UBA6 and USE1 caused increased cell death in FAT10-expressing cells, which may have caused a selective loss of cells with a high FAT10 expression. Nevertheless, the relative quantities of FAT10 conjugates compared with monomeric FAT10 were strongly decreased, both under ectopic and endogenous FAT10 expression. We conclude from these experiments that USE1 is a major E2 enzyme involved in FAT10 conjugation. Whether the few residual putative FAT10 conjugates in siRNA-treated cells are due to incomplete silencing of USE1 or whether other E2 enzymes for FAT10 may exist will need to be addressed in USE1-deficient mice in the future. Thioester bonds between ubiquitin-like modifiers and their E1, E2 or E3 enzymes are normally cleaved by boiling in reducing Laemmli sample buffer, as we have also seen in this study for USE1–ubiquitin and UbcH8–ubiquitin conjugates ( Fig. 3b,c ). It was therefore quite unexpected that the USE1–FAT10 conjugates in transfected HEK293 cells completely resisted boiling in the presence of 10% β-mercaptoethanol and/or 0.5 M dithiothreitol. As formation of this conjugate relied on the active site cysteine of USE1, we reason that USE1 uses activated FAT10 in its active site to form an isopeptide bond between the FAT10 C terminus and one of its 11 lysine residues. This notion was confirmed in cells expressing a lysineless USE1 that also bound to FAT10 but in a reducible manner ( Fig. 5 ). Such an auto-modification of USE1 with FAT10 is reminiscent of E3 ligases of ubiquitin, which also auto-ubiquitylate themselves, and for the auto-SUMOylation reported for Ubc9 [28] . Moreover, E2 enzymes of the ubiquitin system have been shown to monoubiquitylate proteins, which contain different types of ubiquitin interaction domains without the involvement of E3 enzymes [29] . It is hence feasible that USE1 transfers activated FAT10 onto itself in the absence of an E3 enzyme. Along these lines, we investigated whether FAT10 conjugation by USE1 can occur only in cis or also in trans . In Fig. 6 we show that the coexpression of FAT10, together with a catalytically inactive USE1 mutant and wild-type USE1, only led to FAT10 conjugation of the wild-type enzyme, thus demonstrating that USE1 can only FAT10ylate in cis and not in trans . Currently, we are investigating what the consequences of auto-FAT10ylation of USE1 may be. As linkage of FAT10 to long-lived proteins has been shown to target them for degradation by the proteasome in intact cells [16] and in vitro [17] , it is possible that FAT10 self-conjugation by USE1 accelerates the degradation of the modifier-charged E2 enzyme that could constitute a negative feedback mechanism to limit the availability of activated FAT10 in thioester linkage to USE1. Alternatively, FAT10 modification of USE1 could affect its activity as a conjugating enzyme for ubiquitin or FAT10, or it may lead to the association of USE1 with FAT10-binding proteins such as HDAC6 [30] or NUB1L [18] ( Fig. 7 ). 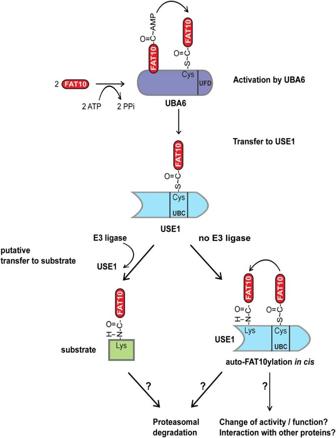Figure 7: Model of the regulation of USE1. FAT10 becomes activated with ATP by the FAT10-specific E1 enzyme UBA6, which adenylates the FAT10 C-terminal carboxyl group, thus forming a FAT10∼AMP intermediate. The intermediate is then transferred onto the active site cysteine of UBA6, where it forms a thioester linkage. By a transthiolation reaction, FAT10 becomes transferred to the active site cysteine of USE1. With the help of an as yet unidentified E3 ligase, FAT10 becomes conjugated through an isopeptide bond to substrates, which might mark them for proteasomal degradation. USE1 undergoes auto-FAT10ylation incisand forms non-reducible isopeptide bonds with FAT10. This could lead to USE1-FAT10 degradation by the proteasome, thus limiting the availability of activated FAT10 in thioester linkage to USE1 in case a putative E3 ligase or substrates are not available. Alternatively, auto-FAT10ylation of USE1 could change its enzymatic properties or mediate the interaction with FAT10-binding proteins such as HDAC6 or NUB1L. UFD, ubiquitin-fold domain; UBC, ubiquitin conjugating enzyme E2 domain. Figure 7: Model of the regulation of USE1. FAT10 becomes activated with ATP by the FAT10-specific E1 enzyme UBA6, which adenylates the FAT10 C-terminal carboxyl group, thus forming a FAT10 ∼ AMP intermediate. The intermediate is then transferred onto the active site cysteine of UBA6, where it forms a thioester linkage. By a transthiolation reaction, FAT10 becomes transferred to the active site cysteine of USE1. With the help of an as yet unidentified E3 ligase, FAT10 becomes conjugated through an isopeptide bond to substrates, which might mark them for proteasomal degradation. USE1 undergoes auto-FAT10ylation in cis and forms non-reducible isopeptide bonds with FAT10. This could lead to USE1-FAT10 degradation by the proteasome, thus limiting the availability of activated FAT10 in thioester linkage to USE1 in case a putative E3 ligase or substrates are not available. Alternatively, auto-FAT10ylation of USE1 could change its enzymatic properties or mediate the interaction with FAT10-binding proteins such as HDAC6 or NUB1L. UFD, ubiquitin-fold domain; UBC, ubiquitin conjugating enzyme E2 domain. Full size image Taken together, we show here that one E1 enzyme (UBA6) specific for the two modifiers, FAT10 and ubiquitin, can transfer both thioester-linked modifiers to one and the same bispecific E2 enzyme (USE1). This is an unprecedented case in the conjugation of ubiquitin family proteins and questions at what stage it will be decided whether a substrate protein will become ubiquitylated or FAT10ylated. The identification of FAT10-specific E3 enzymes may shed light on this interesting question. Primers and constructs The sequences of primers and the description of cloning of expression constructs are available as Supplementary Methods online. Yeast two-hybrid screen Full-length fat10 cDNA was cloned into plasmid pLexA-DIR (pLexA-FAT10) (Dualsystems Biotech) as previously described [18] and used as a bait construct to screen a human thymus cDNA library (Thymus MATCHMAKER cDNA library, Clontech). Briefly, the bait construct was transfected into the yeast strain NMY51 ( MATa his3Δ200 trp1-901 leu2-3,112 LYS2:(lexAop)4-HIS3 ura3:(lexAop)8-lacZ (lexAop)8-ADE2 GAL4 (Dualsystems Biotech)) by a standard LiCl transformation method and the absence of self-activation was tested with an X-Gal filter assay on selection plates lacking tryptophan. For the yeast two-hybrid screen, the human thymus library was transformed into these cells as described by the DUALhybrid kit instructions. Two independent screenings were performed and a total number of 101 clones that grew on selection plates lacking tryptophan, leucine and histidine, supplemented with 1 mM 3-amino-1,2,4-triazole (3-AT) were positively tested by an X-Gal test. For this, yeast cells were grown for 4 days on selection plates lacking tryptophan, leucine and histidine in the presence of 1 mM 3-AT. Whatman filters, which were used to generate replicates of the plates, were frozen in liquid nitrogen, subsequently soaked with PBS containing 100 μg ml −1 X-Gal and incubated at room temperature. Clones that turned blue were grown on new selection plates and subjected to a second X-Gal test. The prey plasmids of the remaining 53 clones were isolated using a standard method with glass beads and were retransformed into NMY51, together with either pLexA-FAT10, pLexA-LaminC or pLexA-p53, to test for bait independency. The identity of the remaining 46 clones was determined by sequencing. Immunoprecipitation HEK293 cells were transfected using FuGene6 (Roche) or TransIT-LT1 transfection reagent (Mirus) as described in the manufacturer's instructions. After 24 h, cells were collected, lysed, and immunoprecipitation was performed as previously described [4] using 30 μl of monoclonal anti-HA-agarose-conjugate HA-7 (Sigma) or EZview Red ANTI-FLAG M2 Affinity Gel (Sigma). Proteins were separated on 4–12% gradient Bis-Tris NuPage SDS gels (Invitrogen) and subjected to western blot analysis using monoclonal anti-polyhistidine–peroxidase-conjugated Ab (clone His-1), monoclonal anti-FLAG (M2), monoclonal anti-HA-7 (all from Sigma) or a ubiquitin-specific, peroxidase-conjugated mAb (clone FK-2, Enzo Life Sciences). For immunoprecipitation of endogenous FAT10, USE1 or FAT10-USE1 conjugate, HEK293T or HEK293 cells were stimulated for 24 h with 200 U ml −1 IFNγ and 400 U ml −1 TNFα (both from Peprotech). Cells were collected, lysed, and immunoprecipitation was performed with a FAT10-reactive mAb ( Supplementary Fig. S3 ) or a USE1-reactive rabbit mAb (kindly provided by B. Amidon, Millennium Pharmaceuticals) bound to protein A sepharose as previously described [4] . Proteins were separated on 4–12% gradient bis-TRIS NuPage SDS gels (Invitrogen) and subjected to western blot analysis using a USE1-specific pAb ( Supplementary Fig. S2 ), a USE1-specific mAb (Millennium Pharmaceuticals), a FAT10-specific pAb [16] or a FAT10-specific mAb ( Supplementary Fig. S3 ). In vitro conjugation assay To generate 35 S-labelled FLAG-His-FAT10, FLAG-His-FAT10ΔGG and HA-ubiquitin proteins, an in vitro transcription and translation T7-coupled reticulocyte lysate system (Promega) was used and the procedures were performed as recommended by the supplier. The translated proteins were purified from the reticulocyte lysate by immunoprecipitation using EZview Red ANTI-FLAG M2 Affinity Gel or anti-HA-sepharose (Sigma) for 2 h at 4 °C. After washing the gel three times, 100 μl reaction mixtures were prepared. Tris pH7.6 (20 mM), 50 mM NaCl, 10 mM MgCl 2 , 5 mM adenosine triphosphate, 1 mM dithiothreitol and 10 U ml −1 inorganic pyrophosphatase were mixed with FLAG-His 6 -FAT10- or HA-ubiquitin bound beads. Where indicated, 250 ng GST-UBA6 and 5 μg His 6 -USE1 of purified proteins were added. The reactions were incubated at room temperature for 30 min, followed by one wash with reaction buffer. A volume of 50 μl of sample buffer containing 4 M urea was added to the beads and incubated at 30 °C for 15 min. Samples were subjected to 8–15% gradient SDS–polyacrylamide gel electrophoresis and detected by autoradiography. USE1 knockdown and real-time PCR HEK293 cells were transfected twice with a pool of four different human USE1-specific siRNAs (Hs_FLJ13855_4, Hs_UBE2Z_5, Hs_UBE2Z_3, Hs_UBE2Z_2, Qiagen) or a pool of four different human UBA6-specific siRNAs (Hs_UBE1L2_1, Hs_UBE1L2_2, Hs_FLJ10808_4, Hs_FLJ10808_2, Qiagen), or with both pools together, or with a control siRNA (AllStars Negative Control siRNA, Qiagen) or single USE1 siRNAs separately, using X-tremeGENE siRNA Transfection Reagent (Roche). On day 1, cells were transfected with a total amount of 400 nM siRNA, and on day 2 with a total amount of 200 nM siRNA. On the third day, cells were transfected with FAT10 expression plasmids pcDNA3.1-3xFLAG-His-FAT10 or pcDNA3.1-3xFLAG-His-FAT10ΔGG, using TransIT-LT1 transfection reagent (Mirus). Cells were collected on the fourth day for anti FLAG immunoprecipitation using EZview Red ANTI-FLAG M2 Affinity Gel (Sigma). Western Blot analysis was performed with a polyclonal anti-USE1 antibody ( Supplementary Fig. S2 ), a polyclonal anti-UBA6 antibody ( Supplementary Fig. S4 , Enzo Life Sciences), a direct peroxidase-labelled anti-FLAG-M2-HRP (Sigma) or as loading control with an antibody directed against β-actin (Abcam). Knockdown of USE1 and UBA6 was verified with real-time RT–PCR on an Applied Biosystems 7900-HT Fast Real-Time PCR Cycler using a QuantiTect SYBRGreen PCR kit (Qiagen) with specific primers for USE1 and UBA6 (QuantiTect Primer Assays Hs_FLJ13855_1_SG and Hs_UBA6_1_SG, Qiagen), and normalized to the expression of GAPDH, which served as housekeeping gene. Specific primers for GAPDH (Hs_99999905_m1) were used with TaqMan Fast Universal PCR Master Mix (both from Applied Biosystems). For siRNA experiments with endogeneous FAT10, FAT10 expression was induced on day 3 with IFNγ/TNFα and on day 4 subjected to an immunoprecipitation using a FAT10 mAb ( Supplementary Fig. S3 ). Immunofluorescence and confocal microscopy Immunofluorescence and confocal microscopy were performed exactly as previously described [30] . Expression and purification of proteins Plasmids pGEX2TKs-UBA6 and pDEST17-USE1 were used for expression of GST-UBA6 and His-USE1. pGEX2TKs-UBA6 was transformed into BL21-CodonPlus(DE3)-RIPL (Stratagene), and pDEST17-USE1 into the strain B834(DE3)pLysS (Novagen). Expression of proteins was induced with 0.1 mM isopropyl- d -thiogalactoside. Purification of GST-UBA6 was carried out using Glutathione-Sepharose 4B (GE Healthcare), as recommended by the supplier. His-USE1 was purified with Protino Ni-IDA Resin (Macherey-Nagel) according to the manufacturer's protocol. How to cite this article: Aichem, A. et al. USE1 is a bispecific conjugating enzyme for ubiquitin and FAT10, which FAT10ylates itself in cis . Nat. Commun. 1:13 doi: 10.1038/ncomms1012 (2010).